Mir-17–92 regulates bone marrow homing of plasma cells and production of immunoglobulin G2c The polycistronic mir-17–92 cluster, also known as oncomir-1 , was previously shown to be essential for early B lymphopoiesis. However, its role in late-stage B-cell differentiation and function remains unexplored. Here we ablate mir-17–92 in mature B cells and demonstrate that mir-17–92 is dispensable for conventional B-cell development in the periphery. Interestingly, mir-17–92 -deficiency in B cells leads to enhanced homing of plasma cells to the bone marrow during T-cell-dependent immune response and selectively impairs IgG2c production. Mechanistically, mir-17–92 directly represses the expression of Sphingosine 1-phosphate receptor 1 and transcription factor IKAROS, which are, respectively, important for plasma cell homing and IgG2c production. We further show that deletion of mir-17–92 could reduce IgG2c anti-DNA autoantibody production and hence mitigate immune complex glomerulonephritis in Shp1-deficient mice prone to autoimmunity. Our results identify important roles for mir-17–92 in the regulation of peripheral B-cell function. B cells and antibodies are central elements of adaptive humoral immunity and critical for host protection. B lymphopoiesis begins with committed haematopoietic stem cells differentiating into pro-B, pre-B and immature B cells in the bone marrow (BM) and cumulates with mature B cells seeding the peripheral lymphoid organs. On activation by foreign antigens, naive B cells undergo terminal differentiation into memory B and antibody-secreting plasma cells (PCs) that provide life-long protection [1] , [2] . B-cell differentiation is governed by a network of transcription factors [3] , [4] . Recently, microRNAs (miRNAs) are shown to exert additional control over B-cell differentiation and function [5] , [6] . MiRNAs are endogenously expressed short non-coding RNAs that fine-tune gene expression at the post-transcriptional level by either promoting the degradation or impeding the translation of target mRNAs [7] , [8] , [9] . A ‘seed region’ of six to eight nucleotides at the 5′ end of a miRNA determines its target specificity [10] . The importance of miRNAs in B-cell biology is highlighted by the drastic defects in mice with global deletion of miRNAs caused by ablating Dicer, a RNAse III endonuclease critical for miRNA processing, in precursor [11] , peripheral mature [12] and activated [13] B cells. When Dicer was deleted at the earliest stage of B-cell maturation using mb-1 Cre, B lymphopoiesis was severely blocked at the pro-B to pre-B-cell transition [11] . This defect was mainly attributed to the absence of mir-17–92 whose seed sequences were enriched in the 3′-untranslated regions (3′UTRs) of mRNAs upregulated in Dicer-deficient pro-B cells [11] . MiR-17–92 , or oncomir-1 , is a polycistronic miRNA cluster that yields six mature miRNAs, including mir-17 , mir-18a , mir-19a , mir-20a , mir-19b and miR-92a . It was first identified as a potent miRNA oncogene on human chromosome 13q31, a region that was amplified in a number of B-cell malignancies [14] , [15] . Overexpression of mir-17–92 in haematopoietic cells significantly accelerated c-Myc induced B-lymphomagenesis in mice [16] and B-cell-specific mir-17–92 transgenic mice developed lymphoma with high penetrance [17] . On the other hand, germline deletion of mir-17–92 compromised early B lymphopoiesis suggesting that mir-17–92 plays essential roles in early B-cell development [18] . Pro-apoptotic BIM was identified as a direct target of mir-17–92 and its upregulation in mutant pro-B cells accounted for the impairment in B-lymphopoiesis [18] . In this study, we deleted mir-17 – 92 in mature B cells using CD19-Cre to examine its role in late-stage B-cell differentiation and function. In contrast to its essential role in early B lymphopoiesis in the BM, mir-17 – 92 -deficency does not perturb conventional B-cell populations in the periphery. Interestingly, during T-cell-dependent (TD) antibody response, there is increased PCs in the BM due to elevated expression of Sphingosine 1-phosphate receptor 1 (S1PR1), which mediates BM homing of PCs [19] . We show that five out of six members of mir-17 – 92 cluster directly target the 3′UTR of S1pr1 and removal of one S1pr1 allele could rebalance S1pr1 expression and normalize the enhanced BM homing phenotype of mir-17 – 92 -deficient PCs. We also reveal that immunoglobulin G2c (IgG2c) production is impaired in the absence of mir-17 – 92 and this defect is due to increased expression of the transcription factor IKAROS, which is important for IgG2c production [20] and directly repressed by mir-92a (ref. 21 ). Furthermore, we demonstrate that mir-17–92 deletion in B cells could reduce IgG2c autoantibody production and attenuate immune complex glomerulonephritis in autoimmune Shp1-deficient mice. Taken together, our findings identify novel roles for mir-17 – 92 in regulating peripheral B-cell function by fine-tuning different target genes. B-cell development in mice lacking mir-17 – 92 in B cells To address the role of mir-17 – 92 in peripheral B cells, we deleted loxP-flanked (floxed) mir-17 – 92 alleles in mice using CD19-Cre that is inefficient with floxed gene deletion in early B cells but mediates efficient gene deletion in mature B lymphocytes [22] . This allows us to bypass the pro-B to pre-B-cell block in mir-17 – 92 germline-deleted mice [18] to investigate its role in the later stages of B-cell maturation and function. Fluorescence-activated sorting (FACS) analyses revealed that the frequency and numbers of pro-B (B220 + CD43 + IgM − ) and pre-B (B220 + CD43 − IgM − ) cells were comparable in the BM of mir-17 – 92 +/+ Cd19 Cre/+ and mir-17 – 92 fl/fl Cd19 Cre/+ (denoted, respectively, as mir-17 – 92 control and mir-17 – 92 bKO thereafter; Fig. 1a , Supplementary Fig. 1a ). Quantitative reverse trancription–PCR (qRT–PCR) analyses indicated that the expression of individual mir-17 – 92 member was not significantly reduced in BM B220 + IgM − pro-B/pre-B cells of mir-17 – 92 bKO mice ( Supplementary Fig. 1b ), suggesting that the almost intact expression of mir-17 – 92 allows for normal progression of early B lymphopoiesis in these mice. However, the expression of individual mir-17 – 92 member was greatly reduced (>80%) in immature (IgM + B220 + ) and recirculating mature (IgM + B220 high(hi) ) B cells in the BM of mir-17 – 92 bKO mice ( Supplementary Fig. 1c,d ) but these two B-cell populations were largely unperturbed ( Fig. 1a ). 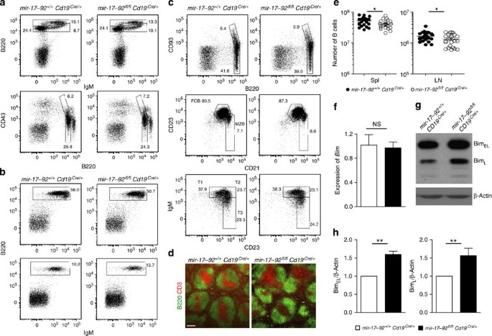Figure 1: Analyses of conventional B cells inmir-17–92bKO mice. (a–c) FACS analyses of B cells in BM (a), spleen (b, upper panel andc) and inguinal lymph nodes (b, lower panel). B220+CD93−splenic B cells were separated into follicular B (FOB: CD23+CD21−) and marginal zone B (MZB: CD23−CD21+) cells, while B220+CD93+cells were divided into transitional I (T1: CD23−IgMhi), II (T2: CD23+IgMhi) and III (T3: CD23+IgMlo) B-cell populations (c). Numbers indicate per cent cells in each gate. (d) Histology of spleens from unchallengedmir-17–92control and bKO mice. B-cell follicles and T-cell areas were identified by B220 (green) and CD3 (red) staining. Scale bar, 100 μm. (e) Enumeration of IgM+B220+B cells in spleen and inguinal lymph nodes. Cell numbers were calculated based on total cell count and their percentage as determined by FACS. (f) Expression ofBimmRNA inmir-17–92bKO B cells. Splenic IgM+B220+B cells frommir-17–92control and bKO mice were examined forBimmRNA expression by qRT–PCR.Bimexpression inmir-17–92bKO B cells was presented relative to that in control B cells. (g) BIM protein expression inmir-17–92bKO B cells. Splenic IgM+B220+B cells were purified and the cell lysates were subjected to western blotting with anti-BIM antibody. The antibody to BIM recognizes two isoforms: BIM extra long (BimEL) and BIM long (BimL). (h) Ratio of BIM to β-actin inmir-17–92control and bKO B cells. The ratio inmir-17–92control B cells was set as 1. Each symbol represents one mouse and horizontal lines indicate the mean. Unpaired two-tailed Student’st-test was used for statistical analyses. NS, not significant; *P<0.05; **P<0.01. Data shown are representative of more than five experiments (a,n=15;b,n=24;c,n=12;d,fandg,n=5). Figure 1: Analyses of conventional B cells in mir-17 – 92 bKO mice. ( a – c ) FACS analyses of B cells in BM ( a ), spleen ( b , upper panel and c ) and inguinal lymph nodes ( b , lower panel). B220 + CD93 − splenic B cells were separated into follicular B (FOB: CD23 + CD21 − ) and marginal zone B (MZB: CD23 − CD21 + ) cells, while B220 + CD93 + cells were divided into transitional I (T1: CD23 − IgM hi ), II (T2: CD23 + IgM hi ) and III (T3: CD23 + IgM lo ) B-cell populations ( c ). Numbers indicate per cent cells in each gate. ( d ) Histology of spleens from unchallenged mir-17 – 92 control and bKO mice. B-cell follicles and T-cell areas were identified by B220 (green) and CD3 (red) staining. Scale bar, 100 μm. ( e ) Enumeration of IgM + B220 + B cells in spleen and inguinal lymph nodes. Cell numbers were calculated based on total cell count and their percentage as determined by FACS. ( f ) Expression of Bim mRNA in mir-17 – 92 bKO B cells. Splenic IgM + B220 + B cells from mir-17 – 92 control and bKO mice were examined for Bim mRNA expression by qRT–PCR. Bim expression in mir-17 – 92 bKO B cells was presented relative to that in control B cells. ( g ) BIM protein expression in mir-17 – 92 bKO B cells. Splenic IgM + B220 + B cells were purified and the cell lysates were subjected to western blotting with anti-BIM antibody. The antibody to BIM recognizes two isoforms: BIM extra long (Bim EL ) and BIM long (Bim L ). ( h ) Ratio of BIM to β-actin in mir-17 – 92 control and bKO B cells. The ratio in mir-17 – 92 control B cells was set as 1. Each symbol represents one mouse and horizontal lines indicate the mean. Unpaired two-tailed Student’s t -test was used for statistical analyses. NS, not significant; * P <0.05; ** P <0.01. Data shown are representative of more than five experiments ( a , n =15; b , n =24; c , n =12; d , f and g , n =5). Full size image The frequency of B220 + IgM + conventional B cells in the spleen and lymph nodes were also indistinguishable between mir-17 – 92 bKO and control mice ( Fig. 1b ). We further observed comparable percentage of follicular B (B220 + CD93 − CD23 + CD21 − ), marginal zone B (B220 + CD93 − CD23 − CD21 + ) and fraction I, II and III transitional B cells in the spleens of mir-17 – 92 bKO and control mice ( Fig. 1c ). B-cell follicles were maintained normally in mir-17 – 92 bKO mice ( Fig. 1d ). The mir-17 – 92 fl/fl alleles were indeed almost completely deleted ( Supplementary Fig. 1e ) and the expression of individual miRNAs significantly reduced (>80%) in various mutant peripheral B-cell populations ( Supplementary Fig. 1f–h ). However, mir-17 – 92 bKO mice had slightly reduced ( ∼ 20%) total B-cell numbers in their spleens and lymph nodes compared with control mice ( Fig. 1e ). As the enhanced expression of pro-apoptotic protein BIM, a known target of mir-17 – 92 , was thought to account for the drastic reduction of mir-17 – 92 -deficient pre-B cells [18] , we examined if the mild reduction of total peripheral B cells in mir-17 – 92 bKO mice could be ascribed to dysregulated BIM expression. Interestingly, Bim mRNA level was comparable between mir-17 – 92 bKO and control B cells ( Fig. 1f ), but BIM protein was enhanced in mir-17 – 92 bKO B cells ( Fig. 1g,h ), suggesting that mir-17 – 92 could modulate BIM expression at the protein level and the subtle decrease in total numbers of mutant peripheral B cells could be due to mildly increased BIM expression. Together, these results suggest that mir-17 – 92 cluster is not essential for conventional B-cell development in the periphery as it is for early B lymphopoiesis. By contrast, both the frequency and total B-cell numbers were found to be reduced in the peritoneal cavities of mir-17 – 92 bKO mice compared with control mice ( Fig. 2a,b ). The reduction was ascribed to decreased B1-a (CD19 + CD43 + CD5 + ) and B1-b (CD19 + CD43 + CD5 − ) cells as their numbers were reduced by approximately seven- and twofold, respectively, whereas conventional B (B2) (CD19 + CD43 − CD5 − ) cells were not significantly affected. These data indicate that mir-17 – 92 is required for B1 cell development or maintenance. 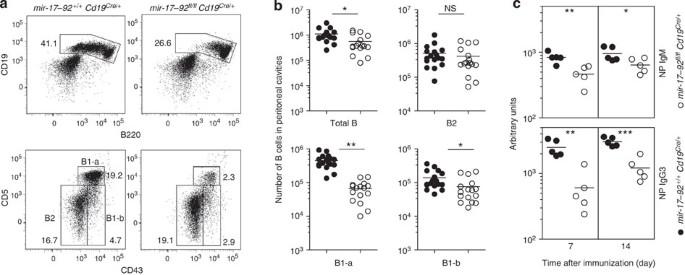Figure 2: Reduced B1 cells and defective TI antibody response inmir-17–92bKO mice. (a) FACS analyses of peritoneal cavity B cells. CD19+B220+B cells were separated into conventional B2 (CD43−CD5−), B1-a (CD43+CD5+) and B1-b (CD43+CD5−) cells. Numbers indicate per cent cells in each gate. (b) Enumeration of various B-cell populations in the peritoneal cavities ofmir-17–92control and bKO mice. (c) Examination of NP-specific IgM and IgG3 antibody inmir-17–92bKO mice. Mice were challenged with TI antigen NP17-Ficoll and sera were collected from immunized mice at day 7 and 14 post immunization. Serially diluted serum samples were subjected to ELISA for the detection of NP-specific IgM and IgG3 antibodies. Cell numbers were calculated based on the total cell count and their percentage as determined by FACS. Unpaired two-tailed Student s t-test was used for statistical analyses. NS, not significant; *P<0.05; **P<0.01, ***P<0.001. Each symbol represents one mouse and horizontal lines indicate the mean. Data shown are representative of 16 (a) and 2 (c) experiments. Figure 2: Reduced B1 cells and defective TI antibody response in mir-17 – 92 bKO mice. ( a ) FACS analyses of peritoneal cavity B cells. CD19 + B220 + B cells were separated into conventional B2 (CD43 − CD5 − ), B1-a (CD43 + CD5 + ) and B1-b (CD43 + CD5 − ) cells. Numbers indicate per cent cells in each gate. ( b ) Enumeration of various B-cell populations in the peritoneal cavities of mir-17 – 92 control and bKO mice. ( c ) Examination of NP-specific IgM and IgG3 antibody in mir-17 – 92 bKO mice. Mice were challenged with TI antigen NP 17 -Ficoll and sera were collected from immunized mice at day 7 and 14 post immunization. Serially diluted serum samples were subjected to ELISA for the detection of NP-specific IgM and IgG3 antibodies. Cell numbers were calculated based on the total cell count and their percentage as determined by FACS. Unpaired two-tailed Student s t-test was used for statistical analyses. NS, not significant; * P <0.05; ** P <0.01, *** P <0.001. Each symbol represents one mouse and horizontal lines indicate the mean. Data shown are representative of 16 ( a ) and 2 ( c ) experiments. Full size image Antibody responses in mir-17 – 92 bKO mice We determined if mir-17–92 is required for B-cell function by examining antibody responses in mutant mice. When immunized with T-cell-independent (TI) antigen 4-hydroxy-3-nitrophenylacetyl (NP) coupled to Ficoll, which elicits IgM and IgG3 antibody production, mir-17 – 92 bKO mice exhibited significantly decreased NP-specific IgM and IgG3 antibody production compared with control mice at day 7 and 14 post immunization ( Fig. 2c ). This defect is consistent with the drastic reduction of B1 cells in these mice, which are the major responders to TI antigens [23] . Thus, mir-17 – 92 is required for TI antibody response. We next examined TD antibody response in mir-17 – 92 bKO mice by challenging them with NP coupled to chicken globulin (NP-CGG). We observed that mir-17 – 92 bKO and control mice produced similar amounts of NP-specific IgM and IgG1 antibodies, the two major antibody isotypes elicited by NP-CGG immunization, at various time points post immunization ( Fig. 3a ). The CD19 + Fas + CD38 − germinal centre (GC) B cells were comparably present in mir-17 – 92 bKO and control mice at day 10 post immunization, and class-switched antigen-specific NIP + IgG1 + (GC) B cells also appeared to be unperturbed in the mutant mice ( Fig. 3b,c ). We further stimulated B cells in vitro with anti-CD40 antibody and interleukin (IL)-4 and found IgG1 class switching to be indistinguishable between mutant and control B cells ( Supplementary Fig. 2a ). These data indicate that mir-17 – 92 is largely not required for GC response and the production of TD class-switched antigen-specific IgG1 antibodies. 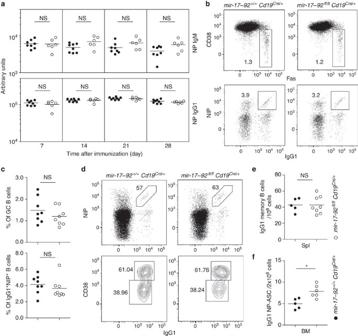Figure 3: TD antibody response inmir-17–92bKO mice. (a) Examination of NP-specific IgM and IgG1 antibody inmir-17–92bKO mice. Mice were challenged with TD antigen NP38-CGG in alum and the sera were collected from immunized mice at the indicated time points. Serially diluted serum samples were subjected to ELISA for the detection of NP-specific IgM and IgG1 antibodies. (b) FACS analysis of GC response inmir-17–92bKO mice at day 10 post immunization. CD19+cells were stained for Fas+CD38−GC B cells (upper panel) and B220+Dump−cells were stained for NP-specific NIP-binding IgG1 B cells (lower panel) from spleens. Numbers indicate per cent cells in each gate. (c) Frequency of GC and NIP+IgG1+B cells in total and B220+Dump−B cells in spleens of immunized mice. (d) FACS analysis of NP-specific IgG1 memory B cells in the spleen of mice 8 weeks after immunization. Splenic cells were stained for B220, IgG1 and CD38 expression and NIP binding after exclusion of dead cells and Dump cells; numbers adjacent to outlined areas indicate the number of cells within the gate among 1 × 106total spleen cells (upper) or per cent cells in each gate (lower). (e) Frequency of NP-specific CD38+IgG1highmemory B cells in spleens ofmir-17–92control and bKO mice as analysed ind. (f) Frequency of long-lived PCs in the BM ofmir-17–92control and bKO mice. NP-specific IgG1 antibody-secreting cells (ASCs) in the BM ofmir-17–92control and bKO mice were determined by ELISPOT assays 8 weeks after immunization and shown as numbers of ASCs per 2 × 106BM cells. Unpaired two-tailed Student'st-test was used for statistical analyses. NS, not significant; *P<0.05. Each symbol represents one mouse and horizontal lines indicate the mean (a,c,e,f). Data shown are representative of two (a,n=6 to 8), six (b) or eight (d) experiments. Figure 3: TD antibody response in mir-17 – 92 bKO mice. ( a ) Examination of NP-specific IgM and IgG1 antibody in mir-17 – 92 bKO mice. Mice were challenged with TD antigen NP 38 -CGG in alum and the sera were collected from immunized mice at the indicated time points. Serially diluted serum samples were subjected to ELISA for the detection of NP-specific IgM and IgG1 antibodies. ( b ) FACS analysis of GC response in mir-17 – 92 bKO mice at day 10 post immunization. CD19 + cells were stained for Fas + CD38 − GC B cells (upper panel) and B220 + Dump − cells were stained for NP-specific NIP-binding IgG1 B cells (lower panel) from spleens. Numbers indicate per cent cells in each gate. ( c ) Frequency of GC and NIP + IgG1 + B cells in total and B220 + Dump − B cells in spleens of immunized mice. ( d ) FACS analysis of NP-specific IgG1 memory B cells in the spleen of mice 8 weeks after immunization. Splenic cells were stained for B220, IgG1 and CD38 expression and NIP binding after exclusion of dead cells and Dump cells; numbers adjacent to outlined areas indicate the number of cells within the gate among 1 × 10 6 total spleen cells (upper) or per cent cells in each gate (lower). ( e ) Frequency of NP-specific CD38 + IgG1 high memory B cells in spleens of mir-17 – 92 control and bKO mice as analysed in d . ( f ) Frequency of long-lived PCs in the BM of mir-17 – 92 control and bKO mice. NP-specific IgG1 antibody-secreting cells (ASCs) in the BM of mir-17 – 92 control and bKO mice were determined by ELISPOT assays 8 weeks after immunization and shown as numbers of ASCs per 2 × 10 6 BM cells. Unpaired two-tailed Student's t -test was used for statistical analyses. NS, not significant; * P <0.05. Each symbol represents one mouse and horizontal lines indicate the mean ( a , c , e , f ). Data shown are representative of two ( a , n =6 to 8), six ( b ) or eight ( d ) experiments. Full size image Increased homing of PCs to BM in mir-17 – 92 bKO mice We also examined in mutant mice the generation of memory B cells and long-lived PCs, which are differentiated through the GC response [24] , [25] . The frequency of NP-specific CD38 + IgG1 high memory B cells was found to be similar in the spleen of mir-17 – 92 bKO and control mice at day 56 post immunization, suggesting that mir-17 – 92 is dispensable for memory B-cell generation and maintenance ( Fig. 3d,e ). However, when long-lived PCs in the BM were examined by enzyme-linked immunospot (ELISPOT) assays, we consistently observed an increase (20–30%) in the frequency of NP-specific IgG1 PCs in mir-17 – 92 bKO compared with control mice ( Fig. 3f ). The increased long-lived PCs in the BM of mir-17 – 92 bKO mice prompted us to examine PCs in detail at early time points after immunization. Strikingly, at day 10 post immunization, the frequency of PCs was ∼ 2.5-fold higher in the BM of mutant mice compared with controls ( Fig. 4a,b ). However, the frequency of splenic PCs from the same mice was not higher but rather reduced ( Fig. 4a,b ). The increased presence of PCs in the BM and decreased frequency of PCs in the spleen of mir-17 – 92 bKO mice was evident as early as day 7 post immunization ( Fig. 4c ). These results suggest that the increased PCs in the BM of immunized mir-17 – 92 bKO mice is not due to exaggerated generation of PCs in the spleen but could be due to the enhanced homing of splenic PCs to the BM during immune response. We further assessed if PC differentiation was perturbed in the absence of mir-17 – 92 by culturing B cells with lipopolysaccharide (LPS) in vitro . After 3 days of LPS stimulation, the percentage of B220 low CD138 + plasmablasts from mir-17 – 92 bKO and control B-cell cultures was comparable ( Supplementary Fig. 2b ), implying that mir-17 – 92 deficiency does not affect PC differentiation per se . Taken together, our data suggest that during an acute antibody response, PC differentiation is normal but homing to the BM is enhanced in the absence of mir-17 – 92 . 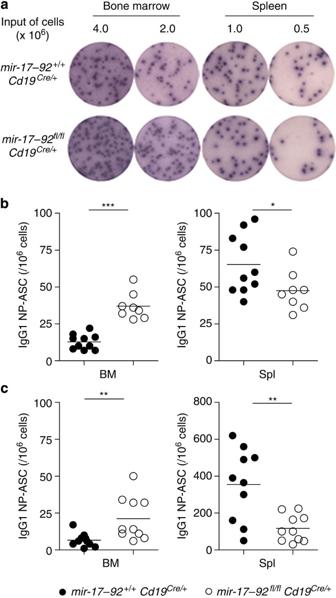Figure 4: Enhanced BM homing of PCs inmir-17–92bKO mice. (a,b) NP-specific IgG1 ASCs in the BM and spleens ofmir-17–92control and bKO mice at day 10 post immunization with NP38-CGG. ASCs in BM and spleens were examined by ELISPOT assays, shown as images of assays (a) and frequency of NP-specific IgG1 ASCs (b). (c) Frequency of NP-specific IgG1 ASCs in the BM and spleens ofmir-17–92control and bKO mice at day 7 after immunization. Unpaired two-tailed Student'st-test was used for statistical analyses. *P<0.05; **P<0.01; ***P<0.001. Each symbol represents one mouse and horizontal lines indicate the mean (b,c). Data shown are representative of eight (a) experiments. Figure 4: Enhanced BM homing of PCs in mir-17 – 92 bKO mice. ( a , b ) NP-specific IgG1 ASCs in the BM and spleens of mir-17 – 92 control and bKO mice at day 10 post immunization with NP 38 -CGG. ASCs in BM and spleens were examined by ELISPOT assays, shown as images of assays ( a ) and frequency of NP-specific IgG1 ASCs ( b ). ( c ) Frequency of NP-specific IgG1 ASCs in the BM and spleens of mir-17 – 92 control and bKO mice at day 7 after immunization. Unpaired two-tailed Student's t -test was used for statistical analyses. * P <0.05; ** P <0.01; *** P <0.001. Each symbol represents one mouse and horizontal lines indicate the mean ( b , c ). Data shown are representative of eight ( a ) experiments. Full size image Mir-17 – 92 directly targets S1pr1 expression in B cells The homing of PCs from secondary lymphoid organs to BM is mainly mediated by sphingosine 1-phosphate (S1P) and chemokine CXCL12 through their engagements of S1PR1 (ref. 19 ) and chemokine-receptor CXCR4 (ref. 26 ), respectively. To understand how mir-17 – 92 modulates BM homing of PCs, we searched for possible targets of mir-17 – 92 using two miRNA target prediction software—TargetScan and MicroCosm, focusing on S1P–S1PR1 and CXCL12–CXCR4 signalling axes, and revealed that S1pr1 is a predicted target gene of mir-17 – 92 with five out of six members of the cluster (namely mir-17 , mir-19a , mir-19b , mir-20a and mir-92a ) targeting it. We next determined if S1pr1 was indeed targeted by mir-17 – 92 . The 3′UTR of S1pr1 contains four predicted binding sites with mir-19a and mir-19b targeting two sites and mir-17 , mir-20a and mir-92a each targeting one site ( Fig. 5a ). A luciferase reporter construct with full-length S1pr1 3′UTR DNA fragment was cloned downstream of firefly luciferase coding sequence and transfected into HEK293 cells together with either the whole mir-17 – 92 cluster or individual relevant miRNAs. We observed significantly reduced luciferase activity with the overexpression of either the whole cluster or individual miRNAs ( Fig. 5b ). We also generated reporter constructs containing individual wild-type (A to D) or mutant (Am to Dm)-binding sites where the DNA sequences complementary to the miRNA seed regions were mutated ( Supplementary Fig. 3 ). When transfected into HEK293 cells with individual miRNAs, the constructs containing wild-type 3′UTR yielded lower luciferase activities compared with the various mutant counterparts ( Fig. 5c ). Thus, our results suggest that S1pr1 is a bona fide target of mir-17 – 92 , with five out of six members directly targeting its 3′UTR at four different sites. 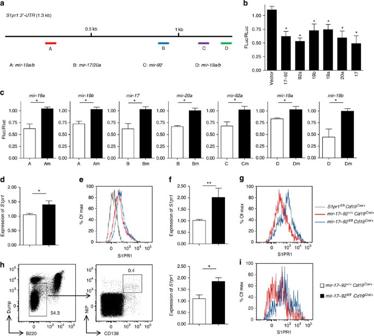Figure 5:Mir-17–92targetsS1pr1in PCs. (a) Schematic representation ofS1p13′UTR and the four predicted binding sites (A to D) formir-17–92. (b,c) Luciferase reporter assay validatingmir-17–92targeting ofS1pr1. HEK293 cells were transfected with full-lengthS1pr13′UTR construct and vectors containingmir-17–92cluster or individualmir-17–92members or control vector (b), or with various WT (a–d) or mutant (Am to Dm)S1p13′UTR constructs and individual miRNAs as depicted (c). Firefly luciferase activity is normalized to renilla luciferase activity (Fluc/Rluc). Results are presented relative to control, set as 1. The Fluc/Rluc for WT 3′UTR constructs (a–d) was presented relative to that for corresponding mutant constructs (Am to Dm). (d,f,h) qRT–PCR analyses ofS1pr1mRNA in sorted resting B220+IgM+B cells (d), LPS-induced CD138+B220low(f) and antigen-specific B220−CD138+NIP+(h, far right panel) plasmablasts. (e,g,i) FACS analyses of S1PR1 on resting B cells (e), LPS-induced (g) and antigen-specific (i) plasmablasts. Mice were immunized twice with NP38-CGG at day 0 and day 28 and sacrificed at day 32. NIP+CD138+plasmablasts were sorted from Dump−B220−spleen cells (h, left and middle panels). Resting B cells fromS1pr1fl/flCd19Cre/+mice were served as a negative control (grey) for S1PR1 staining. Bar graphs represent mean±s.d. (n=3). Expression ofS1pr1inmir-17–92bKO cells (white) was presented relative to that in control cells (black). Unpaired two-tailed Student'st-test was used for statistical analyses. *P<0.05; **P<0.01. Data are representative of three (b–e,g,i) or five (f) experiments. Figure 5: Mir-17 – 92 targets S1pr1 in PCs. ( a ) Schematic representation of S1p1 3′UTR and the four predicted binding sites (A to D) for mir-17 – 92 . ( b , c ) Luciferase reporter assay validating mir-17 – 92 targeting of S1pr1 . HEK293 cells were transfected with full-length S1pr1 3′UTR construct and vectors containing mir-17 – 92 cluster or individual mir-17 – 92 members or control vector ( b ), or with various WT ( a – d ) or mutant (Am to Dm) S1p1 3′UTR constructs and individual miRNAs as depicted ( c ). Firefly luciferase activity is normalized to renilla luciferase activity (Fluc/Rluc). Results are presented relative to control, set as 1. The Fluc/Rluc for WT 3′UTR constructs ( a – d ) was presented relative to that for corresponding mutant constructs (Am to Dm). ( d , f , h ) qRT–PCR analyses of S1pr1 mRNA in sorted resting B220 + IgM + B cells ( d ), LPS-induced CD138 + B220 low ( f ) and antigen-specific B220 − CD138 + NIP + ( h , far right panel) plasmablasts. ( e , g , i ) FACS analyses of S1PR1 on resting B cells ( e ), LPS-induced ( g ) and antigen-specific ( i ) plasmablasts. Mice were immunized twice with NP 38 -CGG at day 0 and day 28 and sacrificed at day 32. NIP + CD138 + plasmablasts were sorted from Dump − B220 − spleen cells ( h , left and middle panels). Resting B cells from S1pr1 fl/fl Cd19 Cre/+ mice were served as a negative control (grey) for S1PR1 staining. Bar graphs represent mean±s.d. ( n =3). Expression of S1pr1 in mir-17 – 92 bKO cells (white) was presented relative to that in control cells (black). Unpaired two-tailed Student's t -test was used for statistical analyses. * P <0.05; ** P <0.01. Data are representative of three ( b – e , g , i ) or five ( f ) experiments. Full size image Modulation of S1PR1 expression in mir-17 – 92 -deficient B cells We proceeded to examine the effect of mir-17 – 92 deficiency on S1PR1 expression in B cells. First, splenic B220 + IgM + B cells were sorted and S1pr1 mRNA was examined by qRT–PCR. We found increased ( ∼ 30%) S1pr1 mRNA level in mir-17 – 92 bKO B cells compared with controls ( Fig. 5d ), which was correlated with a slight increase in cell surface S1PR1 expression as determined by FACS analyses ( Fig. 5e ). We also examined S1pr1 mRNA in sorted CD138 + B220 low plasmablasts differentiated in vitro using LPS and B220 − CD138 + NIP + plasmablasts from the spleens of immunized mice. We found that mir-17 – 92 deficiency led to increase in S1pr1 mRNA ( Fig. 5f,h ), which was corroborated by increased S1PR1 surface levels in the mutant cells ( Fig. 5g,i ). Hence, our data suggest that mir-17 – 92 modulates S1PR1 expression in PCs. Next we investigated if modulating S1PR1 activity or expression in mir-17 – 92 -deficient PCs could influence their homing to BM. It is difficult to test S1P1 function in vitro due to receptor desensitization caused by non-physiological ligand exposure and the inability to model S1P concentration differential that exists across endothelial cells in vivo [27] . Thus, we examined BM homing of PCs in immunized mir-17 – 92 bKO mice in response to different dosages of FTY720 ( Fig. 6a ), a potent S1P1 inhibitor [28] , [29] that impedes the BM homing of PCs from secondary lymphoid tissues [19] . We reasoned that higher S1PR1 expression level in mir-17 – 92 -deficient PCs would render them less sensitive to FTY720 inhibition. Consistent with previous report [19] , when mice were given high dose of FTY720 (3.0 mg kg −1 ), there was hardly any PCs detected in the BM of both mir-17 – 92 control and bKO mice at day 10 post immunization ( Fig. 6b ). Interestingly, when FTY720 dosage was reduced to 1.0 mg kg −1 , NP-specific PCs were found in the BM of mir-17 – 92 bKO but not control mice. When the dosage was further lowered to 0.3 mg kg −1 , we could detect NP-specific PCs in the BM of both mir-17 – 92 control and bKO mice but with the frequency of PCs significantly higher (approximately threefold) in the latter ( Fig. 6b ). These data are consistent with our hypothesis that a higher level of S1PR1 expression in mir-17 – 92 -deficient PCs renders them less sensitive to FTY720 inhibition. 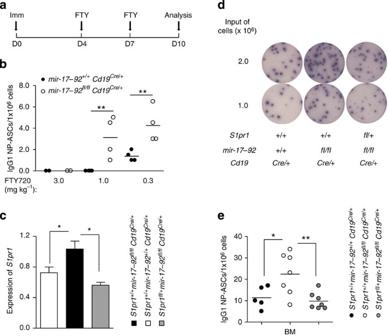Figure 6: Effects of FTY720 inhibition andS1pr1haploinsufficiency onmir-17–92bKO PCs. (a) Timeline of FTY720 treatment and immunization of mice. Mice were immunized with NP38-CGG at day 0 and given FTY720 at different dosages at day 4 and day 7 before analyses at day 10. (b) Frequency of NP-specific IgG1 ASCs in the BM of FTY720-treated mice at day 10 after immunization. (c) ReducedS1pr1expression byS1pr1haploinsufficiency.S1pr1mRNA inmir-17–92fl/flS1pr1fl/+Cd19Cre/+B cells was determined by qRT–PCR and presented relative to that inmir-17–92+/+S1pr1+/+Cd19Cre/+B cells. (d,e) NP-specific IgG1 ASCs in the BM ofmir-17–92+/+S1pr1+/+Cd19Cre/+,mir-17–92fl/flS1pr1+/+Cd19Cre/+andmir-17–92fl/flS1pr1fl/+Cd19Cre/+mice at day 10 post immunization. NP-specific IgG1 ASCs were determined by ELISPOT assays, shown as images of assays (d) and frequency (e). Unpaired two-tailed Student'st-test was used for statistical analyses. *P<0.05. **P<0.01. Each symbol represents one mouse and small horizontal lines indicate the mean (b,e). Bar graphs represent mean±s.d. (n=3). Data are representative of three (c) or five (d) experiments. Figure 6: Effects of FTY720 inhibition and S1pr1 haploinsufficiency on mir-17 – 92 bKO PCs. ( a ) Timeline of FTY720 treatment and immunization of mice. Mice were immunized with NP 38 -CGG at day 0 and given FTY720 at different dosages at day 4 and day 7 before analyses at day 10. ( b ) Frequency of NP-specific IgG1 ASCs in the BM of FTY720-treated mice at day 10 after immunization. ( c ) Reduced S1pr1 expression by S1pr1 haploinsufficiency. S1pr1 mRNA in mir-17 – 92 fl/fl S1pr1 fl/+ Cd19 Cre/+ B cells was determined by qRT–PCR and presented relative to that in mir-17 – 92 +/+ S1pr1 +/+ Cd19 Cre/+ B cells. ( d , e ) NP-specific IgG1 ASCs in the BM of mir-17 – 92 +/+ S1pr1 +/+ Cd19 Cre/+ , mir-17 – 92 fl/fl S1pr1 +/+ Cd19 Cre/+ and mir-17 – 92 fl/fl S1pr1 fl/+ Cd19 Cre/+ mice at day 10 post immunization. NP-specific IgG1 ASCs were determined by ELISPOT assays, shown as images of assays ( d ) and frequency ( e ). Unpaired two-tailed Student's t -test was used for statistical analyses. * P <0.05. ** P <0.01. Each symbol represents one mouse and small horizontal lines indicate the mean ( b , e ). Bar graphs represent mean±s.d. ( n =3). Data are representative of three ( c ) or five ( d ) experiments. Full size image To further determine if increased S1PR1 expression indeed contributed to enhanced PCs homing to the BM in mir-17 – 92 bKO mice, we generated mir-17–92 fl/fl S1pr1 fl/+ Cd19 Cre/+ mice that have one S1pr1 allele specifically deleted in B cells. We reasoned that S1pr1 haploinsufficiency could reduce the elevated expression caused by mir-17 – 92 deficiency and therefore normalize the PC homing phenotype in these mice. First, we examined S1pr1 expression in mir-17 – 92 fl/fl S1pr1 +/+ Cd19 Cre/+ and mir-17 – 92 fl/fl S1pr1 fl/+ Cd19 Cre/+ B cells and found that S1pr1 was reduced ∼ 45% when one S1pr1 allele was ablated ( Fig. 6c ). We next immunized the mice with NP-CGG and examined NP-specific PCs in the BM at day 10 post immunization by ELISPOT assay. As expected, the number of NP-specific IgG1 PCs in the BM of mir-17 – 92 fl/fl S1pr1 +/+ Cd19 Cre/+ mice was increased compared with mir-17 – 92 +/+ S1pr1 +/+ Cd19 Cre/+ mice ( Fig. 6d,e ). Interestingly, when one S1pr1 allele was ablated, the number of NP-specific IgG1 PCs in the BM of mir-17 – 92 fl/fl S1pr1 fl/+ Cd19 Cre/+ mice was reduced compared with mir-17 – 92 fl/fl S1pr1 +/+ Cd19 Cre/+ mice and became similar to that found in mir-17–92 +/+ S1pr1 +/+ Cd19 Cre/+ mice. These results indicate that increased S1PR1 expression indeed contributes to the increased BM homing of PCs in mir-17 –92 bKO mice. Taken together, our data suggest that mir-17 – 92 restrains BM homing of PCs by directly suppressing S1PR1 expression. Impaired IgG2c antibody production in mir-17 – 92 bKO mice During our initial characterization of mir-17 ∼ 92 bKO mice, we found normal levels of IgM, IgG1, IgG3 and IgG2b, but significantly reduced IgG2c antibodies, in the sera of unchallenged mutant mice compared with controls ( Fig. 7a ). It is known that inbred mouse strains such as C57BL/6 and SJL with the Igh-1b allele possess only the gene encoding the IgG2c isotype, whereas BALB/c and 129/Sv strains with the Igh-1a allele express only IgG2a (ref. 30 ). The allele-specific PCR analysis confirmed the presence of IgG2c but not IgG2a gene alleles in mice used in our study ( Supplementary Fig. 4 ), which have been backcrossed to C57BL/6 background for more than 10 generations, and therefore ruled out the possibility that the reduced serum IgG2c in mutant mice was due to different genetic backgrounds. 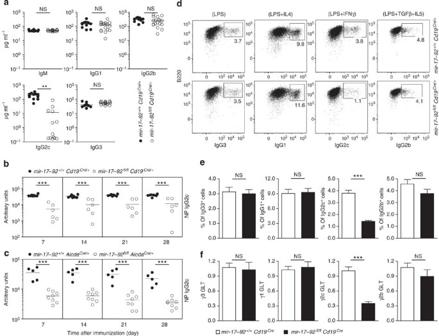Figure 7:MiR-17–92is required for IgG2c production. (a–c) Reduced production of IgG2c antibodies inmiR-17–92-deficient mice. For basal Ig measurement, sera were collected from unchallengedmir-17–92control and bKO mice (a).Mir-17–92control and bKO mice (b) ormir-17–92+/+AicdaCre/+andmir-17–92fl/flAicdaCre/+mice (c) were challenged with NP38-CGG and bled at different days post immunization. Basal Igs (a) or NP-specific IgG2c antibodies (b,c) were examined by ELISA. (d) Defective IgG2c class switching ofin vitro-stimulatedmir-17–92bKO B cells. B cells were cultured for 3 days with LPS, LPS+IL-4, LPS+IFNγ and LPS+TGFβ+IL-5 and class-switched IgG3+, IgG1+, IgG2c+and IgG2b+B cells were analysed by FACS analyses. (e) Percentage of IgG3+, IgG1+, IgG2c+and IgG2b+B cells as culturedin vitroand analysed ind. (f) Reduced IgG2c germline transcript (GLT) in the absence ofmir-17–92. GLTs ofγ3,γ1,γ2candγ2binmir-17–92bKO B cells were determined by qRT–PCR and presented relative to that in control B cells. Unpaired two-tailed Student'st-test was used for statistical analyses. NS, not significant; **P<0.01, ***P<0.001. Each symbol represents one mouse and horizontal lines indicate the mean (a–c). Bar graphs represent mean±s.d. (e,n=10;f,n=5). Data shown are representative of 2 (a,n=15 to 18;b,n=6 to 8;c,n=5 to 8) and 10 (d) experiments. Figure 7: MiR-17 – 92 is required for IgG2c production. ( a – c ) Reduced production of IgG2c antibodies in miR-17 – 92 -deficient mice. For basal Ig measurement, sera were collected from unchallenged mir-17 – 92 control and bKO mice ( a ). Mir-17 – 92 control and bKO mice ( b ) or mir-17 – 92 +/+ Aicda Cre/+ and mir-17 – 92 fl/fl Aicda Cre/+ mice ( c ) were challenged with NP 38 -CGG and bled at different days post immunization. Basal Igs ( a ) or NP-specific IgG2c antibodies ( b , c ) were examined by ELISA. ( d ) Defective IgG2c class switching of in vitro -stimulated mir-17 – 92 bKO B cells. B cells were cultured for 3 days with LPS, LPS+IL-4, LPS+IFNγ and LPS+TGFβ+IL-5 and class-switched IgG3 + , IgG1 + , IgG2c + and IgG2b + B cells were analysed by FACS analyses. ( e ) Percentage of IgG3 + , IgG1 + , IgG2c + and IgG2b + B cells as cultured in vitro and analysed in d . ( f ) Reduced IgG2c germline transcript (GLT) in the absence of mir-17 – 92 . GLTs of γ3 , γ1 , γ2c and γ2b in mir-17 – 92 bKO B cells were determined by qRT–PCR and presented relative to that in control B cells. Unpaired two-tailed Student's t -test was used for statistical analyses. NS, not significant; ** P <0.01, *** P <0.001. Each symbol represents one mouse and horizontal lines indicate the mean ( a – c ). Bar graphs represent mean±s.d. ( e , n =10; f , n =5). Data shown are representative of 2 ( a , n =15 to 18; b , n =6 to 8; c , n =5 to 8) and 10 ( d ) experiments. Full size image We next examined if the production of antigen-specific IgG2c antibodies would be affected during acute antibody response. Interestingly, mir-17 –92 bKO mice had markedly reduced NP-specific IgG2c antibodies at various time points post immunization compared with control mice ( Fig. 7b ). This is in contrast to the normal production of NP-specific IgG1 antibodies in mir-17 –92 bKO mice ( Fig. 3a ). To exclude the possibility that defective IgG2c production in mir-17 –92 bKO mice could be due to the modest reduction of peripheral B-cell numbers in these mice, we generated and analysed mir-17 – 92 fl/fl Aicda Cre/+ mice in which the floxed mir-17 – 92 allele was deleted only in antigen-activated but not naïve B cells ( Supplementary Fig. 5a ). Unchallenged mir-17 – 92 fl/fl Aicda Cre/+ mice had normal B-cell populations in their spleens and lymph nodes compared with mir-17 – 92 +/+ Aicda Cre/+ mice ( Supplementary Fig. 5b,c ). NP-specific IgG1 antibodies were also not drastically affected in mir-17 – 92 fl/fl Aicda Cre/+ mice, especially at later time points post immunization ( Supplementary Fig. 5d ). In contrast, the production of NP-specific IgG2c antibodies was significantly reduced in mir-17 – 92 fl/fl Aicda Cre/+ mice ( Fig. 7c ), suggesting that mir-17 – 92 is indeed important for IgG2c antibody production. To further determine if mir-17 – 92- deficient B cells were intrinsically defective in IgG2c production, we purified B cells from mir-17 –92 bKO and control mice and stimulated them in vitro with LPS+IFN-γ, which induces preferential Ig class switching to IgG2c/2a, and assessed the presence of IgG2c + cells by FACS analysis. After 3 days, mir-17 –92 bKO B-cell culture generated significantly reduced IgG2c + cells ( ∼ 30% of control; Fig. 7d,e ). However, the generation of IgG3 + and IgG1 + B cells after LPS and LPS+IL-4 stimulations, respectively, was comparable between mir-17 –92 bKO and control cultures. The switching to IgG2b in response to LPS+TGFβ+IL-5 stimulation appeared to be reduced but it was not statistically significant ( Fig. 7d,e ). These data suggest that mir-17 – 92 is intrinsically required for IgG2c production in B cells. Mir-17 – 92 regulates GLT and histone acetylation at Cγ2c locus We explored how mir-17 – 92 could regulate IgG2c production. As AID is absolutely required for Ig class switch recombination (CSR), we first assessed if the gene expression of Aicda was affected in mir-17 – 92 -deficent B cells using qRT–PCR. We found comparable Aicda expression between stimulated mir-17 – 92 bKO and control B cells ( Supplementary Fig. 6 ), thus excluding the possibility that the defective IgG2c production was due to dysregulated AID expression. Next we examined germline transcription (GLT) in IgH switch (S) regions, which is important for AID to access ssDNA targets [31] . When germline transcripts for γ3, γ1, γ2c and γ2b in various B-cell cultures were determined by qRT–PCR, we detected marked reduction in γ2c GLT in mir-17 – 92 bKO cells stimulated with LPS+IFNγ compared with controls, whereas γ3, γ1 and γ2b GLT levels were largely comparable between mutant and control cells ( Fig. 7f ). Chromatin remodelling is required for many DNA-directed processes, such as transcription, recombination and replication. Acetylation (Ac) on amino-terminal tails of histone H3 and H4 at S regions has been shown to be important for Ig GLT and CSR [32] , [33] . We therefore performed chromatin immunoprecipitation (ChIP)-qPCR to assess the acetylation of histone H3 (H3Ac) and H4 (H4Ac) at the S region and Cγ2c I exon of LPS+IFNγ-treated B cells using specific antibodies. When measured by ChIP–qPCR, mutant cells had lower H3Ac levels were lower at the S region and Cγ2c I exon compared with control cells at 48 h after LPS+IFNγ stimulation ( Fig. 8a ), correlating with decreased IgG2c GLT in mutant B cells ( Fig. 7f ). Consistent with the normal IgG1 GLT ( Fig. 7f ), H3Ac levels at Sγ1/Iγ1 loci were comparable between mutant and control B cells stimulated with LPS+IL-4 ( Fig. 8b ). We also examined H4Ac at Cγ2c S region, which is known to reflect AID accessibility and activity at S regions and important for CSR [32] . We showed that H4Ac level at Sγ2c was lower in LPS+IFNγ-stimulated mir-17 – 92 bKO cells compared with similarly treated control cells ( Fig. 8c ), indicating reduced AID accessibility at Sγ2c region of mutant cells. However, H4Ac level at the Sγ1 region was comparable in LPS+IL-4-treated mir-17 – 92 bKO and control cells ( Fig. 8d ). Taken together, these results suggest that mir-17 – 92 deficiency affects chromatin remodelling at Cγ2c/2a locus and consequently, GLT, AID accessibility and CSR. 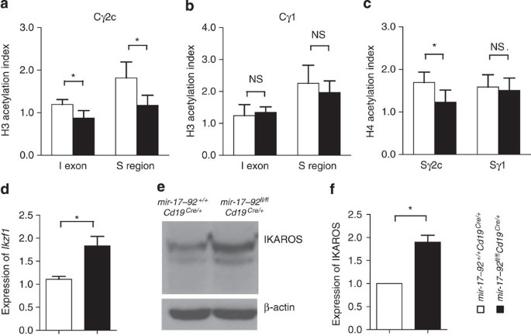Figure 8: Reduced histone acetylation at Cγ2c locus and increased IKAROS expression in B cells lackingmiR-17–92. (a) Reduced histone H3 acetylation atCγ2cin the absence ofmir-17–92bKO.Mir-17–92control and bKO B cells were stimulated with LPS+IFNγ for 2 days and subjected to ChIP with anti-AcH3 or control antibodies. (b) Comparable histone H3 acetylation atCγ1inmir-17–92bKO control B cells.Mir-17–92control and bKO B cells were stimulated with LPS+IL-4 for 2 days and subjected to ChIP with anti-AcH3 or control antibodies. (c) Impaired histone H4 acetylation atSγ2cin the absence ofmir-17–92bKO.Mir-17–92control and bKO B cells were stimulated with LPS+IFNγ or LPS+IL-4 for 2 days and subjected to ChIP with anti-AcH4 or control antibodies. ChIP and input DNA was quantified by qPCR. Percentage of AcH3 and AcH4 enrichment was calculated as ChIP DNA relative to 10% input DNA. The AcH3 or AcH4 index was shown as the ratio of per cent histone acetylation enrichment at I exon or S region to that atGapdhpromoter region. (d–f) Increased IKAROS expression inmir-17–92-deficient B cells.Mir-17–92control and bKO B cells were stimulated with LPS+IFNγ for 2 days. The levels ofIkzf1mRNA (d) and IKAROS protein (e) were determined by qRT–PCR and western blotting, respectively. The ratio of IKAROS protein to β-actin inmir-17–92control and bKO B cells was calculated (f). Bar graphs represent mean±s.d. (n=3 fora–d;n=5 forf). Data are representative of five (e) experiments. Unpaired two-tailed Student'st-test was used for statistical analyses. NS, not significant; *P<0.05. Figure 8: Reduced histone acetylation at Cγ2c locus and increased IKAROS expression in B cells lacking miR-17 – 92 . ( a ) Reduced histone H3 acetylation at Cγ2c in the absence of mir-17 – 92 bKO. Mir-17 – 92 control and bKO B cells were stimulated with LPS+IFNγ for 2 days and subjected to ChIP with anti-AcH3 or control antibodies. ( b ) Comparable histone H3 acetylation at Cγ1 in mir-17 – 92 bKO control B cells. Mir-17 – 92 control and bKO B cells were stimulated with LPS+IL-4 for 2 days and subjected to ChIP with anti-AcH3 or control antibodies. ( c ) Impaired histone H4 acetylation at Sγ2c in the absence of mir-17 – 92 bKO. Mir-17 – 92 control and bKO B cells were stimulated with LPS+IFNγ or LPS+IL-4 for 2 days and subjected to ChIP with anti-AcH4 or control antibodies. ChIP and input DNA was quantified by qPCR. Percentage of AcH3 and AcH4 enrichment was calculated as ChIP DNA relative to 10% input DNA. The AcH3 or AcH4 index was shown as the ratio of per cent histone acetylation enrichment at I exon or S region to that at Gapdh promoter region. ( d – f ) Increased IKAROS expression in mir-17 – 92 -deficient B cells. Mir-17 – 92 control and bKO B cells were stimulated with LPS+IFNγ for 2 days. The levels of Ikzf1 mRNA ( d ) and IKAROS protein ( e ) were determined by qRT–PCR and western blotting, respectively. The ratio of IKAROS protein to β-actin in mir-17 – 92 control and bKO B cells was calculated ( f ). Bar graphs represent mean±s.d. ( n =3 for a – d ; n =5 for f ). Data are representative of five ( e ) experiments. Unpaired two-tailed Student's t -test was used for statistical analyses. NS, not significant; * P <0.05. Full size image Mir-92a directly targets Ikzf1 and regulates IgG2c production As miRNAs negatively regulate gene expression, we hypothesized that mir-17 – 92 could target negative regulator(s) of IgG2c CSR that likely also regulates chromatin remodelling. Hence, the absence of mir-17 – 92 would lead to the derepression of negative regulator(s) and result in reduced IgG2c production. It was previously shown that IKAROS deficiency led to increased and ectopic switching to IgG2c/2a (ref. 20 ). IKAROS was also showed to maintain repressive chromatin at Cγ2c/2a and suppress GLT, AID accessibility and CSR of IgG2a/2c (ref. 20 ). More recently, Ikzf1 , the gene encoding IKAROS, was demonstrated to be directly targeted by mir-92a in T cells [21] . Given that mir-17 – 92 -deficient B cells exhibited reduced GLT and hypoacetylation of histone at Sγ2c region, we postulated that mir-17 – 92 likely regulated IgG2a/2c switching by modulating IKAROS expression in activated B cells. We found that Ikzf1 was indeed targeted by mir-17 – 92 or mir-92a but not by other members of the cluster using luciferase reporter assays ( Supplementary Fig. 7 ). We demonstrated that mir-17 – 92 -deficient B cells had higher ( ∼ 60%) Ikzf1 mRNA levels than control cells when treated with LPS+IFNγ ( Fig. 8d ). Consistent with increased Ikzf1 mRNA, the protein level of IKAROS was also enhanced in stimulated mutant cells as determined by western blotting ( Fig. 8e,f ). These results together indicate that mir-17–92 directly targets Ikzf1 and modulates IKAROS expression in B cells. We next asked if elevated IKAROS expression could account for the defective IgG2c production in mir-17 – 92 -deficient B cells. We used short interfering RNA (siRNA) to knock-down IKAROS in the mir-17 – 92 -deficient cells with nucleofection, which can efficiently transfect activated B cells in vitro ( Supplementary Fig. 8 ). Western blotting analyses showed that IKAROS protein level was noticeably reduced in mutant B cells transfected with Ikzf1 -targeting siRNA compared with control siRNA ( Fig. 9a ). More importantly, Ikzf1 -silenced mutant B cells had increased IgG2c class switching compared with non-silenced counterparts ( Fig. 9b,c ). We further demonstrated that introduction of mir-92a mimics but not others could enhance IgG2c production in mir-17 – 92 -deficient and control B cells ( Fig. 9d ). Taken together, our data suggest that mir-92a from mir-17 – 92 cluster directly represses IKAROS expression and regulates IgG2c production. 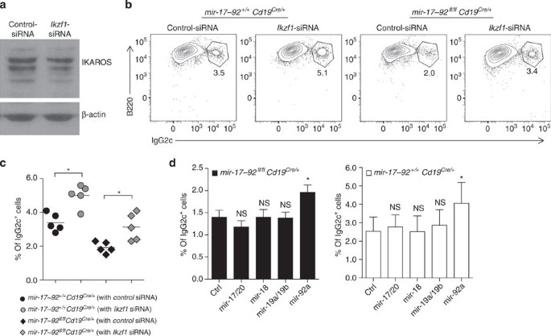Figure 9:MiR-92modulates IgG2c antibody production via targetingIkzf1. (a)Ikzf1knockdown inmir-17–92bKO B cells by siRNA.Mir-17–92bKO B cells were stimulated with LPS+IFNγ and nucleotransfected with control orIkzf1-targeting siRNA and IKAROS protein expression was examined by western blotting. (b,c) Increased IgG2c+B cells byIkzf1knock-down. LPS+IFNγ-stimulatedmir-17–92control and bKO B cells were nucleotransfected with control orIkzf1-targeting siRNAs. The presence of IgG2c+B cells was assessed by FACS analyses (b) and their percentages were depicted inc. (d) Increased IgG2c+B cells resulting frommir-92overexpression.Mir-17–92control and bKO B cells were stimulated with LPS+IFNγ and nucleotransfected with control or various miRNA mimics as indicated. Bar graphs represent mean±s.d. (d,n=5). Each symbol represents one mouse and horizontal lines indicate the mean (c). Data are representative of three (a) or five (b) experiments. Unpaired two-tailed Student'st-test was used for statistical analyses. NS, not significant; *P<0.05. Figure 9: MiR-92 modulates IgG2c antibody production via targeting Ikzf1 . ( a ) Ikzf1 knockdown in mir-17 – 92 bKO B cells by siRNA. Mir-17 – 92 bKO B cells were stimulated with LPS+IFNγ and nucleotransfected with control or Ikzf1 -targeting siRNA and IKAROS protein expression was examined by western blotting. ( b , c ) Increased IgG2c + B cells by Ikzf1 knock-down. LPS+IFNγ-stimulated mir-17 – 92 control and bKO B cells were nucleotransfected with control or Ikzf1 -targeting siRNAs. The presence of IgG2c + B cells was assessed by FACS analyses ( b ) and their percentages were depicted in c . ( d ) Increased IgG2c + B cells resulting from mir-92 overexpression. Mir-17 – 92 control and bKO B cells were stimulated with LPS+IFNγ and nucleotransfected with control or various miRNA mimics as indicated. Bar graphs represent mean±s.d. ( d , n =5). Each symbol represents one mouse and horizontal lines indicate the mean ( c ). Data are representative of three ( a ) or five ( b ) experiments. Unpaired two-tailed Student's t -test was used for statistical analyses. NS, not significant; * P <0.05. Full size image Mir-17 – 92 deficiency attenuates murine autoimmunity IgG2c/2a is the most prevalent autoantibody isotype found in murine lupus [34] , [35] . These autoantibodies bind self DNA and ribonucleoproteins to form immune complexes that cause tissue damage. The systemic autoimmunity in mir-17–92 -transgenic mice [36] , [37] and selective IgG2c defect in mir-17 – 9 fl/fl Cd19 Cre/ + mice led us to explore if mir-17 – 92 ablation could attenuate B-cell-mediated autoimmunity. Hence, we introduced mir-17 – 92 deficiency into Ptpn6 fl/fl Cd19 Cre/+ mice that had Shp1 tyrosine phosphatase deleted in B cells and developed autoimmunity resembling that of human lupus [38] . Compared with age-matched Ptpn6 +/+ mir-17 – 92 +/+ Cd19 Cre/+ control mice, 10-week-old Ptpn6 fl/fl mir-17 – 92 +/+ Cd19 Cre/+ mice manifested increased sera titres of IgM and IgG2c antibodies reactive to single-stranded (ss) and double-stranded (ds) DNA. Interestingly, sera titres of anti-ssDNA and anti-dsDNA IgM antibody were diminished by 50–60% in Ptpn6 fl/fl mir-17 – 92 fl/fl Cd19 Cre/+ mice ( Fig. 10a,b ), which could be due to the reduction of IgM antibody-producing B1 cells resulting from mir-17 – 92 -deficiency ( Fig. 2 ). Strikingly, anti-DNA antibodies of the IgG2c isotype, which were abundantly present in Ptpn6 fl/fl mir-17 – 92 +/+ Cd19 Cre/+ mice, were significantly reduced in Ptpn6 fl/fl mir-17 – 92 fl/fl Cd19 Cre/+ mice. Immunofluorescence staining of renal sections ( Fig. 10c ) revealed the presence of prominently coarse granular and segmental IgG depositions in the mesangium of the glomeruli of Ptpn6 fl/fl mir-17 – 92 +/+ Cd19 Cre/+ mice, which was indicative of immune complex glomerulonephritis. Interestingly, the amount of IgG immune complex deposition was significantly reduced in the kidneys of Ptpn6 fl/fl mir-17 – 92 fl/fl Cd19 Cre/+ mice ( Fig. 10c,d ). These results suggest that the ablation of mir-17 – 92 could potentially suppress IgG2c autoantibody production and therefore alleviate symptoms of systemic autoimmunity in mice. 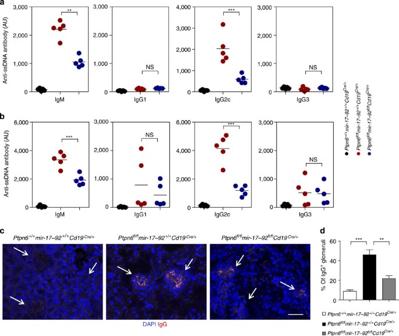Figure 10: Ablation ofmir-17–92in B cells attenuates autoimmunity in Shp1-deficient mice. (a,b) Sera titres of anti-ssDNA (a) and anti-dsDNA (b) antibodies of 10-week-oldPtpn6+/+mir-17–92+/+Cd19Cre/+,Ptpn6fl/flmir-17–92+/+Cd19Cre/+andPtpn6fl/flmir-17–92fl/flCd19Cre/+mice. Serum samples were assayed by ELISA for IgM, IgG1, IgG2c and IgG3 anti-DNA antibodies. (c,d) Immunofluorescence staining of renal sections of 10-week-old mice of different genotypes as indicated. Anti-mouse IgG (red) antibody was used to reveal IgG immune complexes in glomeruli (indicated by white arrows) and DAPI (blue) was used to stain DNA of renal cells (c). Scale bar, 100 μm. The percentages of IgG-staining positive glomeruli among∼100–120 glomeruli examined per kidney were calculated (d). Each symbol represents one mouse and small horizontal lines indicate the mean. Bar graphs represent mean±s.d. (d,n=5). Data are representative of two (a,b) and five (c) experiments. Unpaired two-tailed Student'st-test was used for statistical analyses. NS, not significant; **P<0.01; ***P<0.001. Figure 10: Ablation of mir-17 – 92 in B cells attenuates autoimmunity in Shp1-deficient mice. ( a , b ) Sera titres of anti-ssDNA ( a ) and anti-dsDNA ( b ) antibodies of 10-week-old Ptpn6 +/+ mir-17 – 92 +/+ Cd19 Cre/+ , Ptpn6 fl/fl mir-17 – 92 +/+ Cd19 Cre/+ and Ptpn6 fl/fl mir-17 – 92 fl/fl Cd19 Cre/+ mice. Serum samples were assayed by ELISA for IgM, IgG1, IgG2c and IgG3 anti-DNA antibodies. ( c , d ) Immunofluorescence staining of renal sections of 10-week-old mice of different genotypes as indicated. Anti-mouse IgG (red) antibody was used to reveal IgG immune complexes in glomeruli (indicated by white arrows) and DAPI (blue) was used to stain DNA of renal cells ( c ). Scale bar, 100 μm. The percentages of IgG-staining positive glomeruli among ∼ 100–120 glomeruli examined per kidney were calculated ( d ). Each symbol represents one mouse and small horizontal lines indicate the mean. Bar graphs represent mean±s.d. ( d , n =5). Data are representative of two ( a , b ) and five ( c ) experiments. Unpaired two-tailed Student's t -test was used for statistical analyses. NS, not significant; ** P <0.01; *** P <0.001. Full size image We examined the role of mir-17 – 92 in late-stage B-cell differentiation and function by ablating it using CD19-cre. We show that mir-17 – 92 is not absolutely required for conventional B-cell maturation in the periphery in contrast to its essential role in early B lymphopoiesis. However, we unveil two novel roles for mir-17 – 92 in peripheral B cells, namely the modulation of PC homing to the BM and selective regulation of IgG2c production. We further identify S1PR1 and IKAROS as direct physiological targets of mir-17 – 92 responsible for these two outcomes. Previous studies have postulated that mir-17 – 92 could largely account for Dicer’s function in early B-lymphoiesis by targeting BIM [11] , [18] . Here we demonstrate that mir-17 – 92 is largely dispensable for the maturation of conventional B cells in the periphery, suggesting that it plays a more important role in early B-lymphoiesis than in peripheral B-cell maturation. However, we demonstrate that mir-17 – 92 is required for B1 cell development and TI immune response. We also show that BIM protein but not mRNA level is increased in mir-17 – 92 -deficient B cells and could account for the modestly decreased total peripheral B cells in mir-17 – 92 bKO mice. Previous studies of mir-17 – 92 -deficient or -overexpressing B cells [11] , [39] have demonstrated either enhanced or decreased BIM protein expression in mutant B cells, but Bim mRNA level was not examined in those studies. Our results suggest that mir-17 – 92 regulation of BIM mainly occurs at the protein level. In contrast to the absolute requirement for Dicer in GC response [13] , mir-17 –92 bKO mice have normal NP-specific IgM and IgG1 antibody production and unperturbed GC during TD antibody response, suggesting that miRNAs other than mir-17 – 92 are important for these processes. In support of this view, a previous miRNA deep-sequencing study has shown that mir-17 – 92 family members are not amongst the most highly expressed miRNAs in GC B cells [40] . Interestingly, we show that mir-17 – 92 is important for modulating PC homing to BM where survival niches are provided for their long-term persistence [41] , [42] , [43] . We show that five out of six members of mir-17 – 92 cluster target the 3′UTR of S1pr1 at four different sites and the absence of mir-17 – 92 leads to higher S1pr1 expression in PCs. It is possible that S1pr1 could be synergistically and simultaneously targeted by these five miRNAs in PCs. The enhanced BM homing of PCs in mir-17 –92 bKO mice can be normalized by removing one copy of S1pr1 gene. Thus, our data suggest that mir-17 – 92 -mediated fine-tuning of S1PR1 expression is another means to control BM homing of PCs, and this insight could be useful for the development of miRNA-based drugs to interfere with PC homing to BM survival niches in PC-related diseases such as multiple myeloma and autoimmunity. The mir-17 – 92 -mediated modulation of S1PR1 expression and enhanced homing of PCs in mutant mice raise the possibility that the slightly decreased peripheral B cells in mutant mice might be due to increased egress of B cells from secondary lymphoid organs into circulation. However, our analyses showed that the distribution of naïve B cells in blood and secondary lymphoid organs was comparable between mir-17 – 92 bKO and control mice ( Supplementary Fig. 9 ), suggesting that the mildly increased S1PR1 level in mutant naïve B cells does not significantly shift the equilibrium distribution of B cells in favour of blood. The noticeable homing phenotype of mutant PCs but not naïve B cells could be due to the different expression levels of mir-17 – 92 , which is upregulated in PCs ( Supplementary Fig. 10 ), or the differential expression of other S1PR1-targeting miRNAs in these cells. We also show that mir-17 – 92 deficiency in B cells impairs IgG2c antibody production, which is accompanied by abnormal GLT and chromatin remodelling at Cγ2a/2c locus. We further demonstrate that mir-17 – 92 can inhibit the expression of IKAROS, the transcription factor known to maintain repressive chromatin at Cγ2C/2a, and therefore suppress transcription, AID accessibility and CSR of IgG2a/2c [20] . It was recently demonstrated that IKAROS expression in B cells could be modulated by the transcription factor IRF5 (ref. 44 ). Thus, our current study uncovers a post-transcriptional layer of IKAROS regulation by miRNAs. Interestingly, in IKAROS hypomorphic mice that have 10-fold less IKAROS protein than wild-type mice [20] , the production of IgG2b was also enhanced. However, in our study, we did not observe a significant change in IgG2b production in mir-17 – 92 -deficient B cells. This could be due to the mild (approximately twofold) increase in IKAROS expression in these cells. In agreement with this viewpoint, IgG2b was also not affected in IRF5-deficent B cells, which manifested modest changes in IKAROS expression [44] , [45] . It is possible that IgG2c/2a CSR is more sensitive to subtle changes in IKAROS levels than that of other Ig isotypes. Another interesting finding from our study is that mir-17 – 92 deletion in B cells can significantly reduce the amount of pathogenic IgG2c anti-DNA antibodies in autoimmune Shp1-deficient mice. In addition, IgG immune complex glomerulonephritis in Shp1-deficient mice could be attenuated by mir-17 – 92 deficiency. Murine IgG2c/IgG2a and its analogue isotype IgG1 in humans are the most prevalent and potent Ig isotypes found in autoimmune diseases [46] , [47] , [48] , [49] . Therefore, our results suggest that mir-17 – 92 could be a possible target for therapeutic intervention by providing an avenue to control pathogenic IgG2c autoantibody production in lupus. Mice Mir-17 – 92 fl/fl , S1pr1 fl/fl , Ptpn6 fl/fl and Cd19 Cre/+ mice were obtained from The Jackson Laboratory. Aicda Cre/+ mouse was generated and described previously [13] and maintained in C57BL/6 background. Mir-17 – 92 fl/fl mice were backcrossed >10 generations into C57BL/B background before intercrossing with Cd19 Cre/+ and Aicda Cre/+ mice to generate mir-17 – 92 fl/fl Cd19 Cre/+ and mir-17 – 92 fl/fl Aicda Cre/+ mice. Genotyping of IgG2a and IgG2c alleles was performed by PCR using allele-specific primers as described [30] previously. Mice of 10 to 16 weeks old of both genders were used according to the protocols approved by the Institutional Animal Care and Use Committees (IACUCs) based on guidelines from the National Advisory Committee on Laboratory Animal Research (NACLAR) of Singapore. Immunization and FTY720 administration Mice were immunized intraperitoneally with 100 μg NP-CGG 38 (Biosearch Technologies) precipitated in Imject alum (Pierce, Biotechnology). For the in vivo inhibition of S1PR1, immunized mice were given various doses (3.0, 1.0 and 0.3 mg kg −1 ) of FTY720 (Cayman Chemical) twice by intraperitoneal injection. Flow cytometry Cells were harvested from BM, spleen, inguinal lymph nodes, peritoneal cavities and peripheral blood of mice and treated with Fc-block and stained with biotin- or fluorescent-labelled monoclonal antibodies (mAbs) as described [13] . The following mAbs were from BD Pharmingen or as specified: fluorescein isothiocyanate (FITC) anti-Fas (Cat. No: 554257), FITC anti-CD19 (Cat. No: 553785), FITC anti-IgG1 (Cat. No: 553443), FITC anti-CD21 (Cat. No: 553818), FITC-IgM (Cat. No: 553408); phycoerythrin (PE) anti-Fas (Cat. No: 554258), PE anti-CD138 (Cat. No: 553714), PE anti-B220 (Cat. No: 553090), PE anti-CD5 (Cat. No: 553023), PE anti-CD93 (ebioscience, Cat. No:12–5892); biotinylated (bio-) anti-CD38 (Cat. No: 553762), bio-anti-IgM (Cat. No: 553406), bio-anti-IgD (Cat. No: 553506), bio-anti-CD138 (Cat. No: 553717), bio-anti-CD43 (Cat. No: 553269), anti-CD62L (Cat. No: 553149), bio-anti-Thy1.2 (Cat. No: 553002), bio-anti-CD3 (Cat. No: 663060), bio-anti-Gr-1 (Cat. No: 553125), bio-anti-F4/80 (Biolegend; Cat. No:108404), bio-anti-CD5 (Cat. No:553019), bio-anti-Ter119 (Cat. No: 553612), bio-anti-DX5 (Cat. No: 553856), bio-anti-NK1.1 (Cat. No: 553163), bio-anti-CD93 (Cat. No: 550434), bio-anti-IgG3 (Cat. No: 553401), bio-anti-IgG1 (Cat. No: 553441), bio-anti-IgG2c (Cat. No:553504) and bio-anti-IgG2b (Cat. No: 553393); allophycocyanin (APC) anti-CD19 (Cat. No: 550992), APC anti-CD38 (ebioscience; Cat. No:17–0381), APC-Cy7 anti-B220 (Cat. No: 552094), APC Cy7anti-CD19 (Cat. No: 557655). Biotin conjugates were visualized with Streptavidin-conjugated peridinin chlorophyll protein-cyanine 5.5 (PerCP-Cy5.5; Cat. No:551419), Streptavidin-conjugated APC (Cat. No: 554067) or APC-Cy7 (Cat. No: 554063). Fluorescein-labelled Peanut agglutinin (PNA) and 4′,6-Diamidino-2-phenyindole (DAPI) were purchased from Sigma-Aldrich. PE-labelled NIP-BSA (Biosearch Technologies) were prepared using R-PE labelling kit-SH (Dojindo). All the antibodies were used in 1:100 dilution except specified elsewhere. Dead cells were excluded electronically using DAPI. Exclusion staining (Dump) for antigen-specific GC B cells or PCs included anti-IgM, anti-IgD, anti-CD138, anti-CD3, anti-Th1.2, anti-Gr-1, anti-F4/80, anti-Ter119, anti-Dx5, anti-NK1.1, anti-AA4.1 and anti-CD5 mAbs; or anti-IgD, anti-IgM, anri-CD4, anti-CD8, anti-F4/80 and anti-Gr-1 mAbs. Cell surface staining of S1PR1 was performed using rat anti-S1PR1 antibody (R&D System) [50] . In brief, cells were stained with rat anti-S1PR1 (5 μg/ml) followed by donkey anti-rat IgG biotin and streptavidin-APC-Cy7. Data were collected on LSR II flow cytometer (BD Pharmingen) and analysed with Flowjo (Treestar). Cell sorting and qRT–PCR For cell isolation, pro-B/pre-B (IgM − B220 + ), immature B (IgM + B220 + ) and mature B (IgM + B220 hi ) cells from BM and transitional B (B220 + AA4.1 + ), follicular B (B220 + AA4.1 − CD23 + CD21 − ), marginal zone B (B220 + AA4.1 − CD23 − CD21 + ) and total B (IgM + B220 + ) cells from spleens of unchallenged mice and GC B (CD19 + CD38 − Fas + ), non-GC B (CD19 + CD38 + Fas − ) cells and PCs (Dump − B220 lo/− CD138 + NIP + ) from spleens of immunized mice were sorted directly into Trizol LS with FACSAria (BD Pharmingen). Total RNA was prepared from sorted cells and subjected to cDNA synthesis with reverse transcriptase using random hexamers as primers (Research Instruments). Platinum SYBR Green Supermix (Life Technologies) was used in quantitative real-time PCR (qRT–PCR) for Bim , S1pr1 and Ikzf1 using primers as follow: Bim (forward: 5′-CGACAGTCTCAGGAGGAACC-3′, reverse: 5′-CAATGCCTTCTCCATACCAGA-3′), S1pr1 (forward: 5′-GAGTCCTGCGGACGCAGCTT-3′, reverse: 5′-AGCCAGGTCAGCGAGCAATCC-3′) and Ikzf1 (forward: 5′-GGATCATTCTTGGCCCCCAAA-3′, reverse: 5′-ACCCTCATCGACATCCATTGT-3′). TaqMan MicroRNA system (Life Technologies) was used for miRNA quantification. GLT levels for γ3 , γ1 , γ2c and γ2b were determined as described [20] previously. Immunofluorescence histology Splenic and renal sections of 8 μm thickness were prepared from tissues frozen in Tissue-Tek (Sakura) as described previously [13] . After blocking, sections were stained at room temperature for 30 min with a cocktail of antibodies and mounted with CYTOSEAL 60 (Electron Microscopy Sciences) and analysed on a FV1000 confocal microscope (Olympus). ELISA and ELISPOT assay Sera were collected from unchallenged or immunized mice on various days. Total or NP-specific antibodies of various isotypes in sera were measured via enzyme-linked immunosorbent assay (ELISA). The relative titres of NP-specific serum antibodies are shown as the relative of dilutions that give absorbance reading within the linear range of the assay [51] . The frequency of NP-specific IgG1 antibody-secreting cells was determined by ELISPOT assay [13] . Plasmid construction and luciferase reporter assay Mir-17 , mir-18a , mir-19a , mir-19b , mir-20a , mir-92a and mir-17 – 92 cluster were cloned into MSCV retroviral vector. The 3′UTR fragments of mouse S1pr1 and Ikzf1 with predicted binding sites for individual miRNAs and their mutants were amplified from genomic DNA and inserted into pmirGLO plasmid (Promega) and confirmed by sequencing. For luciferase reporter assay, HEK 293 cells were plated into 48-well plates at 1 × 10 5 cells per well 16 h before transfection. pmirGLO (0.2 μg) reporter plasmid containing the S1pr1 and Ikzf1 3′UTR fragments or their mutants and 0.2 μg different miRNA-expressing plasmids were transfected into each well using Lipofectamine 2000 transfection reagent (Invitrogen) in triplicate. Luciferase assays were performed 48 h after transfection using the Dual-Luciferase Reporter Assay System (Promega) on a SpectraMax Luminescence Microplate Reader (Molecular Devices). Luciferase activity was expressed as ratio between firefly and renilla luciferase activities. Cell culture and nucleofection of B cells Splenic B cells were purified with anti-CD43 mAb-coupled magnetic beads using magnetic-activated cell sorting negative selection protocol (Miltenyi Biotech, Bergisch Gladbach, Germany). Cells were stimulated for 3 days with 10 μg ml −1 LPS (Sigma) in DMEM supplemented with the necessary additives. IL-4 (10 ng ml −1 ), IL-5 (5 ng ml −1 ), IFNγ (10 ng ml −1 ) and TGFβ (2 ng ml −1 ) from R&D Systems were used to induce preferential Ig class switching to various isotypes. For nucleofection, purified B cells were stimulated with 10 μg ml −1 LPS and 10 ng ml −1 IFNγ overnight and transfected with siRNA or miRNA mimics from Life Technologies using P4 Primary Cell 4D-Nucleofector X Kit on an Amaxa 4D-nucleofector (Lonza). Transfected cells were recultured and analysed 48 h later. Western blotting Cells were lysed and protein concentrations were determined as described previously [52] . Equal amount of proteins was loaded and subjected to SDS–polyacrylamide gel electrophoresis, transferred and blotted with specific antibodies. BIM-specific antibody (C34C5) was from Cell Signalling. The IKAROS-specific antibody (M20) was from Santa Cruz. Western blot images shown in Figs 1 , 8 and 9 have been cropped for presentation. Full-sized images are presented in Supplementary Fig. 11 . ChIP–qPCR ChIP was performed using EZ-ChIP kit (Millipore) according to the manufacturer’s protocol. In brief, 1 × 10 7 stimulated B cells were crosslinked in 1% formaldehyde. Chromatin was sonicated to 500–1,000 bp using Misonix Sonicator 3000 Ultrasonic Cell Disruptor (QSonica). Sonicated chromatin was precleared with Protein G Agarose and subsequently subjected to immunoprecipitation with anti-H3Ac, anti-H4Ac or control antibodies (Millipore). One per cent of the precleared chromatin was saved as input. Protein/DNA complexes were eluted and reverse crosslinked to free DNA, which was further purified using spin columns (Millipore). The input DNA was diluted 10 times. Two μl of DNA samples was analysed by qPCR using Iγ1 , Sγ1 , Iγ2c , Sγ2c and Gapdh primers [20] , [53] . The acetylation index was calculated described previously [20] . Statistics Unpaired two-tailed Student’s t -test was used for statistical analyses. How to cite this article: Xu, S. et al. Mir-17–92 regulates bone marrow homing of plasma cells and production of immunoglobulin G2c. Nat. Commun. 6:6764 doi: 10.1038/ncomms7764 (2015).